Water-walled microfluidics for high-optical finesse cavities In submerged microcavities there is a tradeoff between resonant enhancement for spatial water and light overlap. Why not transform the continuously resonating optical mode to be fully contained in a water microdroplet per se ? Here we demonstrate a sustainable 30-μm-pure water device, bounded almost completely by free surfaces, enabling >1,000,000 re-circulations of light. The droplets survive for >16 h using a technique that is based on a nano-water bridge from the droplet to a distant reservoir to compensate for evaporation. More than enabling a nearly-perfect optical overlap with water, atomic-level surface smoothness that minimizes scattering loss, and ∼ 99% coupling efficiency from a standard fibre. Surface tension in our droplet is 8,000 times stronger than gravity, suggesting a new class of devices with water-made walls, for new fields of study including opto-capillaries. Liquids have served microcavity research from Ashkin’s studies on optical resonances in levitating droplets [1] to recent optofluidic [2] resonators [3] . Droplets can provide an optical quality factor ( Q ) in proximity to the limit restricted by water absorption and radiation loss [4] . However, water microdrops [5] quickly vaporize due to their large area/volume ratio. The current state of the art in optofluidic resonators [3] , [6] , [7] includes single-use droplets in experiments with a pulse laser [5] , water in pipettes [8] , toroids in water [9] , [10] , [11] , [12] , submerged spheres in water [13] , a stream of microdroplet dye lasers [14] , water droplets in oil [15] and water glycerol on a hydrophobic surface [12] and microfluidic optomechanics [16] . Modern techniques used to perform measurements on solid resonators can be utilized for these resonators as well. Among them are cancelling frequency drifts in the resonator [10] and in the pump [11] , cavity-enhanced spectroscopy [7] , [14] , [17] , broad-band spectroscopy using frequency combs [18] , and recently, exploiting ring-up for ultrafast spectroscopy [19] . In their inherent essence, microcavities confine multiple optical passes. Accordingly, and with several close descriptions encountered in literature, the major goodness-of-fit parameters of such resonators are their smallness, 1/ V m (ref. 20 ), where V m is the volume of the optical mode, their optical quality factor, Q , and the optical intensity at the region of interest [20] . Water walls are used in various applications [21] including reactions at a gas-liquid interface [22] . Here we fabricate a stable spheroidal shape water-walled droplet around a cylindrical stem ( Fig. 1 ). Light can circulate in this droplet near its interface, and when the circumference is an integer number of wavelengths, an optical resonance known as a whispering-gallery mode is formed. There are many advantages to water-walled devices enveloped in air. A maximal contrast between air and the water-core results in a minimal radiation loss, allowing for tight confinement (1/V m ; ref. 4 ). In addition, air is so transparent that the droplet’s Q can be limited by water absorption only. Last, optical intensity is almost totally contained in the water near the interface with air. Therefore, thermal capillary waves [23] can interact with resonantly enhanced light near the interface [24] . 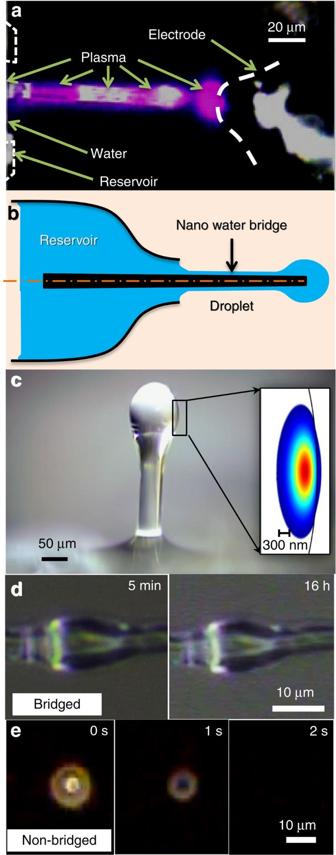Figure 1: Droplet sustainer. (a) A silica stem is plasma treated to modify its hydrophilicity. A water microdroplet is then formed near the stem’s end ((b) right) while in fluidic contact with a water reservoir ((b) left) via a nano water bridge covering the stem ((b) centre). (c) Micrograph of the drop together with its calculated mode (inset). (d) The bridged droplet maintained its shape for 16 h. (e) Control group: evaporation of a non-bridged droplet on a plate. Vertical and horizontal configurations were equivalent here, since gravity is negligible when compared with surface tension. Figure 1: Droplet sustainer. ( a ) A silica stem is plasma treated to modify its hydrophilicity. A water microdroplet is then formed near the stem’s end (( b ) right) while in fluidic contact with a water reservoir (( b ) left) via a nano water bridge covering the stem (( b ) centre). ( c ) Micrograph of the drop together with its calculated mode (inset). ( d ) The bridged droplet maintained its shape for 16 h. ( e ) Control group: evaporation of a non-bridged droplet on a plate. Vertical and horizontal configurations were equivalent here, since gravity is negligible when compared with surface tension. Full size image Fabrication of the droplet sustainer We will now describe our method for sustaining the water walls of a microfluidic device ( Supplementary Movie 1 ). As one can see in Fig. 1b,c , a nanoscale water bridge extends from the droplet all the way to a practically unlimited reservoir that replenishes it. Total compensation for evaporation is achieved by designing the hydrophilicity and geometry of our solid surfaces, to enable this bridge; while bearing in mind that water, from energy consideration, prefers to minimize the product of interfacial-tension and area. As will be explained in more details in ( Supplementary Fig. 1 , Supplementary Methods , Supplementary note 1-2 ), a wet-plasma treated [25] ( Fig. 1a ) cylindrical stem holds the microdroplet ( Fig. 1b,c ) while in fluidic contact with the water bridge ( Fig. 1b centre). The micrograph of our sustainer presents a droplet ( Fig. 1c ), where light can circumferentially circulate along an equatorial line and may form an optical whispering-gallery resonance. On need, water can surround the full length of the stem ( Fig. 1c ) including the formation of a droplet at its end. The existence of the water bridge is confirmed by touching it with a dry object, and watching the object absorb liquid. The droplet endures perturbations such as holding it (with its sustainer) in a hand and walking with it to another set-up. The droplet also survives touch by a 1-μm tapered fibre. In fact, the taper broke in such tests while the droplet lived on. This is expected since surface tension governs at small scales. To put it into perspective, surface tension in our device is >8,000 times stronger than gravity as defined by its Eötvös number ( Supplementary Note 3 ), meaning that such droplets might even withstand high accelerations. While regular droplets at these scales quickly vaporize ( Fig. 1e and Supplementary Movie 2 ), our microfluidic device was sustained for >16 h ( Fig. 1d ); when we had to interfere and cut the experiment, to continue to the next study. Characterization of water droplet resonator In the following, we will demonstrate our claim to high- Q optical resonances in this sustainable water droplet. We use a tapered fibre [12] , [15] , [26] , [27] to evanescently couple light in and out of the droplet ( Fig. 2a ). We scan the laser wavelength over a region that contains one or more of its resonances. We then deduce the optical quality factor of our micro-droplet resonator from the measured optical linewidth (Δ λ ) with the formula Q = λ /Δ λ . 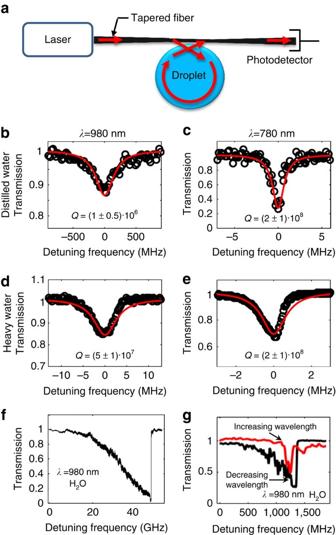Figure 2: Optical resonances in micro water droplets. (a) Experimental set-up (b–e) Monitoring resonator transmission while scanning the wavelength through resonance provides the linewidth. (f) Coupling efficiency close to 99% was measured at critical coupling conditions. (g) Thermal asymmetry of the resonance linewidth measured from two consequented scans. The droplet’s diameter was between 20 and 40 μm. The water is high-purity deionized water (18 MΩ cm−1) and the heavy water is deuterium oxide 99.9 atom % D (item# 151882–100G from Sigma-Aldrich). The taper to resonator distance is 900 nm at the under-coupled regime (Fig. 3b–e) and 700 nm at the critically coupled regime (f). This distance between the taper and resonator was estimated based on the input from the droplet positioning system (P-611.3 NanoCube, Physik Instrumente, PI). Figure 2: Optical resonances in micro water droplets. ( a ) Experimental set-up ( b – e ) Monitoring resonator transmission while scanning the wavelength through resonance provides the linewidth. ( f ) Coupling efficiency close to 99% was measured at critical coupling conditions. ( g ) Thermal asymmetry of the resonance linewidth measured from two consequented scans. The droplet’s diameter was between 20 and 40 μm. The water is high-purity deionized water (18 MΩ cm −1 ) and the heavy water is deuterium oxide 99.9 atom % D (item# 151882–100G from Sigma-Aldrich). The taper to resonator distance is 900 nm at the under-coupled regime ( Fig. 3b–e ) and 700 nm at the critically coupled regime ( f ). This distance between the taper and resonator was estimated based on the input from the droplet positioning system (P-611.3 NanoCube, Physik Instrumente, PI). Full size image The quality factor was tested on heavy and distilled water droplets at the red and near infrared as shown in Fig. 2b–e . Both distilled and heavy water supports an optical finesse over a million at 780 nm. As seen when diving in the ocean, blue light penetrates water much deeper than red. Thus, 480 nm light will enable one, or maybe even two, orders of magnitude improvement in our measured finesse. Still, even at 780 nm, with an almost complete optical mode overlap with water, the product of finesse and mode penetration in water in our system is >1,000 times higher than other devices. This said, finesse higher than ours was demonstrated using solid devices [28] . Our quality factors ( Fig. 2c,e ) suggest an upper limit for scattering losses in our system. Scattering, including from Brownian capillary waves [24] , might occur in our system; yet, they attenuate light by <0.0001, cm −1 . By bringing the taper closer to the droplet we establish critical coupling. As a result, transmission at resonance drops to almost zero ( Fig. 2f ), indicating that the coupling efficiency to our devise is ∼ 99% (ref. 27 ). Contrary to common solids, the thermal broadening [29] is seen here ( Fig. 2g ) while scanning towards the shorter wavelengths. This is expected since the thermal coefficient of refractive index for water is negative. Linewidth narrowing ( Fig. 2g ) was observed when scanning toward the longer wavelength exhibiting thermal asymmetry similar to what is readily seen in solid-state resonators [29] . Increasing the optical input power up to 1 mW results no changes in the resonator and its modal properties when compared with a solid-state resonator. Characterization of the resonance stability and tenability Too measure the stability of the resonance during evaporation and subsequent replenishment, we perpetually scan our laser frequency through resonance while monitoring transmission and tracking the resonance ( Fig. 3a ). We find deviation of 0.3 Å in radius and 0.6 GHz in resonance frequency as calculated from the s.d. of 16 measurements that span over a 0.08-s period. We again monitor the resonance; however, this time we apply voltage to the droplet. As one can see in Fig. 3b , a 10 GHz frequency drift (corresponding to a 5 Å increase in the droplet radius) was observed on increasing the voltage by 10 V. In this regard, it was suggested that hydration shells, including droplets, prefer negative charges [30] , which can explain the pulling of the droplet toward the positive electrode. 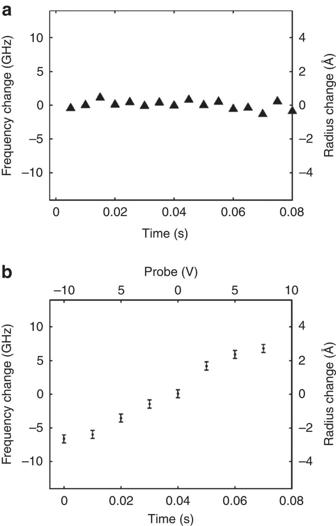Figure 3: Experimental results. (a) Monitoring the droplet size through its resonance frequency reveals a s.d. of 0.3 Å in radius during a 0.08 s period. Parameters here are similar with the ones inFig. 2cwhere the resonance frequency is revealed from the centre of the best-fitting Lorentzian (red line,Fig. 2c). (b) Controlling the water-droplet size and its resonance frequency by applying an external voltage. Parameters are similar to (a) except for an electrode here that was located 300 μm from the droplet. The error bars in (b) represents the s.d. when voltage was not applied (a). We note that the water reservoir is always grounded. Figure 3: Experimental results. ( a ) Monitoring the droplet size through its resonance frequency reveals a s.d. of 0.3 Å in radius during a 0.08 s period. Parameters here are similar with the ones in Fig. 2c where the resonance frequency is revealed from the centre of the best-fitting Lorentzian (red line, Fig. 2c ). ( b ) Controlling the water-droplet size and its resonance frequency by applying an external voltage. Parameters are similar to ( a ) except for an electrode here that was located 300 μm from the droplet. The error bars in ( b ) represents the s.d. when voltage was not applied ( a ). We note that the water reservoir is always grounded. Full size image As for Q variation, we monitored no Q degradation over time, even after using the same set-up for a few days without washing it. Our method worked with every type of water that we tried. This includes the purest water that we could find, as well as the dirtiest water that exhibited a quality factor near 10,000. Applicability of liquid-walled resonators to other fluids is evident by the fact that we could successfully excite similar resonances in non-evaporating liquids such as silicone oil and paraffin. Organic liquids (such as acetone) that we tested benefitted from a very-good adhesion to the stem. However, at this preliminary stage we could not find an organophobic material for the reservoir. In conclusion, devices bounded by water-air interfaces can host optical resonances at their edges. Until today, the fast evaporation of the entire device challenged such experiments. This technology stopper is mitigated here by establishing a nano water bridge that feeds the device. This enables water walls almost all-over microfluidic devices at room pressure and temperature, with no controller, no feedback loop and no additives to the water. How to cite this article: Maayani, S. et al . Water-walled microfluidics for high optical finesse cavities. Nat. Commun. 7:10435 doi: 10.1038/ncomms10435 (2016).